A fungal protease allergen provokes airway hyper-responsiveness in asthma Asthma, a common disorder that affects >250 million people worldwide, is defined by exaggerated bronchoconstriction to inflammatory mediators including acetylcholine (ACh), bradykinin and histamine—also termed airway hyper-responsiveness. Nearly 10% of people with asthma have severe, treatment-resistant disease, which is frequently associated with immunoglobulin-E sensitization to ubiquitous fungi, typically Aspergillus fumigatus ( Af ). Here we show that a major Af allergen, Asp f13 , which is a serine protease, alkaline protease 1 (Alp 1), promotes airway hyper-responsiveness by infiltrating the bronchial submucosa and disrupting airway smooth muscle (ASM) cell-extracellular matrix (ECM) interactions. Alp 1-mediated ECM degradation evokes pathophysiological RhoA-dependent Ca 2+ sensitivity and bronchoconstriction. These findings support a pathogenic mechanism in asthma and other lung diseases associated with epithelial barrier impairment, whereby ASM cells respond directly to inhaled environmental allergens to generate airway hyper-responsiveness. In asthma, chronic lung inflammation due to the immune response to inhaled allergens leads to desquamation of the respiratory epithelium, increased bronchial smooth muscle mass and mucous gland hypertrophy [1] , [2] . However, the mechanisms by which such airway ‘remodelling’ brings about enhanced contraction of airway smooth muscle (ASM) cells to pro-contractile ligands are poorly understood [3] . Intraperitoneal immunization of mice with a diverse array of allergens including ovalbumin (OVA), house dust mite (HDM) or Aspergillus fumigatus ( Af ) followed by respiratory mucosal challenge induces what is termed as ‘allergic sensitization’: expansion of allergen-specific T helper type 2 (T H 2) cells, synthesis of allergen-specific immunoglobulin-E (IgE) and production of cytokines in lung including interleukin-4 (IL-4), IL-5 and IL-13. These events result in allergic inflammation including goblet cell metaplasia, increased mucous production, leukocyte infiltration (predominantly eosinophils) and collagen deposition in the bronchial submucosa [4] , [5] , [6] , [7] . Protease activity is a common and important feature of many allergens capable of inducing asthma. A secreted protease of Aspergillus oryzae ( Ao ) was shown to elicit T H 2 immunity and allergic inflammation in mice through proteolytic cleavage of fibrinogen. Fibrinogen cleavage products can act as Toll-like receptor 4 ligands on respiratory epithelial cells, innate lymphoid cells and macrophages to elicit cytokine production and upregulation of mucin genes that promote the asthma phenotype [8] . Serine protease allergens can both activate and impair respiratory epithelial functions. An alkaline serine protease from the allergenic fungus Penicillium citrinum ( Pen c13 ) induced proinflammatory cytokine release in airway epithelial cells through activation of coagulation factor II (thrombin) receptor and coagulation factor II-like receptor 2 (F2R and F2RL1, previously known as protease-activated receptors (PAR) 1 and 2) [9] . Both Pen c 13 and a serine protease component of the ubiquitous mold Alternaria alternata induce respiratory epithelial barrier dysfunction through altered cell–cell junctions and actin cytoskeletal rearrangements [10] , [11] . Induction of allergic sensitization and airway hyper-responsiveness (AHR) in mice by allergens generally requires priming with both the allergen and an adjuvant at sites distant from the lung. However, short-term respiratory mucosal exposure of mice to protease-containing allergens such as Af or Ao may evoke AHR without prior remote priming with allergen and adjuvant [12] . Inhalation of proteolytically active Ao , but not its protease-inactive counterpart, elicited nearly equivalent AHR in the presence or absence of OVA, which did not correlate strictly with the magnitude of allergic inflammatory response (IgE response and airway eosinophilia). Likewise, the purified, secreted Af protease, which itself is poorly immunogenic [13] , induced AHR in the presence of OVA despite recruiting markedly fewer airway eosinophils to the lung than OVA plus crude Af allergen. These results suggest that proteolytic activity of certain allergens, while not sufficient to elicit AHR in the absence of lung inflammation, nonetheless contribute to AHR through mechanisms independent of allergic sensitization. Whether allergens have a direct and pathogenic impact on ASM contraction in asthma has not been explored. Here we investigate the hypothesis that lung epithelial destruction associated with asthma permits penetrance of allergen components into the bronchial submucosa to promote ASM contraction. We detect an Af -derived protease (Alp 1) in the bronchial smooth muscle layer of human subjects with asthma and allergen-challenged mice but not in control subjects or naïve mice, and we provide a potential mechanism by which Alp 1 induces a pro-contractile phenotype of ASM cells. Af protease activity promotes AHR Proteolytic enzymes secreted by Af cause epithelial desquamation and have an integral function in tissue invasiveness [14] , [15] . We found that a commercially available and clinically used Af extract had readily detectable protease activity, which was abolished by heat inactivation or preincubation with inhibitors of serine proteases (phenylmethylsulfonyl fluoride or antipain), but not cysteine proteases (E-64) ( Fig. 1a ). To determine the relative importance of Af protease activity for the induction of AHR, we sensitized and challenged mice with either native or heat-inactivated (HI)- Af allergen extracts and measured total lung resistance ( R L ) in anesthetized mice following methacholine inhalation. As expected, mice challenged with untreated Af had significantly increased R L compared with naïve mice ( Fig. 1b ). Mice challenged with HI- Af had significantly reduced R L values compared with mice that received untreated Af . However, native or HI- Af induced comparable sensitization, as evidenced by equivalent peribronchial inflammation, goblet cell metaplasia ( Fig. 1c ) and total cell counts in bronchoalveolar lavage fluid ( Fig. 1d ), although the composition of BAL fluid differed modestly between the two groups. Challenge with HI- Af elicited slightly fewer airway eosinophils and a greater influx of neutrophils than did challenge with untreated Af ( Fig. 1e ). These results suggest that Af protease activity also contributes to AHR through mechanisms distinct from the inflammatory response. 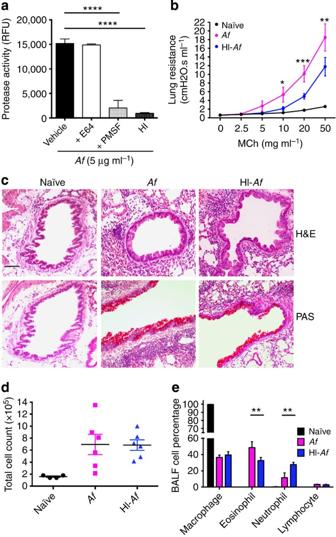Figure 1:Afprotease activity promotes AHR. (a) Protease activity in crudeAfextracts incubated with vehicle alone, PMSF (serine protease inhibitor, 250 μM), E-64 (cysteine protease inhibitor, 10 μM) or heat-inactivated (HI)-Afwas determined as described in Methods. Bar graph shows mean±s.e.m. of three independent experiments (****P<0.0001, one-way analysis of variance (ANOVA)). (b) Lung resistance (RL) in response to aerosolized methacholine (MCh) was measured in naïve,Afor HI-Af-sensitized and challenged BALB/c WT mice 24 h after the final challenge. Data inb–eare represented as mean±s.e.m. of four to six mice per group measured in a single experiment (*P=0.04, **P=0.001, ***P=0.0006, two-way ANOVA, comparingAfversus HI-Af). (c) Peribronchial infiltration and goblet cell metaplasia of paraffin-embedded mouse lungs were evaluated by using haematoxylin/eosin and Periodic acid–Schiff staining, respectively (Scale bar, 100 μm, original magnification, 10 × ). (d) Total cell counts and (e) differentials were assessed in BALF cytospin preparations. (**P<0.01 two-way ANOVA). Figure 1: Af protease activity promotes AHR. ( a ) Protease activity in crude Af extracts incubated with vehicle alone, PMSF (serine protease inhibitor, 250 μM), E-64 (cysteine protease inhibitor, 10 μM) or heat-inactivated (HI)- Af was determined as described in Methods. Bar graph shows mean±s.e.m. of three independent experiments (**** P <0.0001, one-way analysis of variance (ANOVA)). ( b ) Lung resistance ( R L ) in response to aerosolized methacholine (MCh) was measured in naïve, Af or HI- Af -sensitized and challenged BALB/c WT mice 24 h after the final challenge. Data in b – e are represented as mean±s.e.m. of four to six mice per group measured in a single experiment (* P =0.04, ** P =0.001, *** P =0.0006, two-way ANOVA, comparing Af versus HI- Af ). ( c ) Peribronchial infiltration and goblet cell metaplasia of paraffin-embedded mouse lungs were evaluated by using haematoxylin/eosin and Periodic acid–Schiff staining, respectively (Scale bar, 100 μm, original magnification, 10 × ). ( d ) Total cell counts and ( e ) differentials were assessed in BALF cytospin preparations. (** P <0.01 two-way ANOVA). Full size image Af induces lung slice airway contraction To determine whether Af could elicit bronchoconstriction without prior allergic sensitization, we pre-treated precision-cut lung slices (PCLS) extracted from lungs of naïve mice with Af extracts for 24 h and visualized airway contraction in response to carbachol (an ACh analogue similar to methacholine). Compared with PCLS incubated with vehicle alone, lung slices pre-treated with Af had spontaneously narrowed airways at baseline ( Fig. 2a ) and displayed a dose-dependent increase in carbachol-mediated bronchoconstriction ( E max : vehicle=31.99±2; Af (5 μg ml −1 )=53.06±3.5; Af (10 μg ml −1 )=66.64±3.7; P <0.0001; EC 50 unchanged) ( Fig. 2b ). In contrast, vehicle- and Af -pre-treated PCLS had equivalent contraction in response to KCl, which depolarizes cell membranes through a voltage-gated Ca 2+ channel [16] , [17] ( Fig. 2c ). Together, these findings indicated that Af specifically and independently augments G protein-coupled receptor (GPCR)-mediated bronchoconstriction in the absence of prior allergen sensitization and challenge. 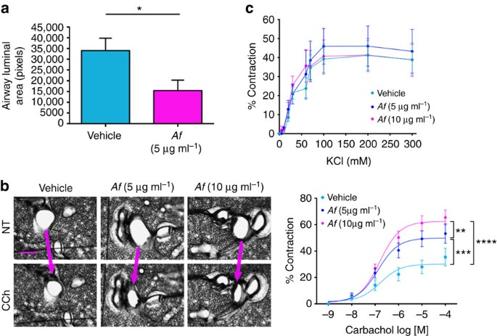Figure 2:Afinduces bronchoconstriction in PCLS. Mouse lung slices were pre-treated with vehicle orAf(5 or 10 μg ml−1) for 24 h. (a) Bright field images of airways in PCLS treated with vehicle orAf(5 μg ml−1) were obtained and used to calculate baseline airway luminal areas as per the Methods. (mean±s.e.m. of 26–45 airways evaluated in 2–3 experiments; *P=0.03,t-test). (b) Left panel: bright field images were obtained before (NT) and 4 min after carbachol (CCh, 100 μM) stimulation. Scale bar, 300 μm; original magnification, 5 × . Arrows denote contracting airways. Right panel: slices were stimulated with increasing concentrations of CCh, and percent contraction was calculated based on the airway luminal area. Data are expressed as mean±s.e.m. of three independent experiments (23–25 airways per group) fitted to a curve using the least-squares fit method.Emaxwas compared between groups by extra sum-of-squareFtest (**P<0.01, ***P<0.001, ****P<0.0001, two-way analysis of variance). (c) PCLS were prepared as inaand stimulated with the indicated concentrations of KCl. Data are represented as mean±s.e.m. of two independent experiments (9–15 airways per group). Figure 2: Af induces bronchoconstriction in PCLS. Mouse lung slices were pre-treated with vehicle or Af (5 or 10 μg ml −1 ) for 24 h. ( a ) Bright field images of airways in PCLS treated with vehicle or Af (5 μg ml −1 ) were obtained and used to calculate baseline airway luminal areas as per the Methods. (mean±s.e.m. of 26–45 airways evaluated in 2–3 experiments; * P =0.03, t -test). ( b ) Left panel: bright field images were obtained before (NT) and 4 min after carbachol (CCh, 100 μM) stimulation. Scale bar, 300 μm; original magnification, 5 × . Arrows denote contracting airways. Right panel: slices were stimulated with increasing concentrations of CCh, and percent contraction was calculated based on the airway luminal area. Data are expressed as mean±s.e.m. of three independent experiments (23–25 airways per group) fitted to a curve using the least-squares fit method. E max was compared between groups by extra sum-of-square F test (** P <0.01, *** P <0.001, **** P <0.0001, two-way analysis of variance). ( c ) PCLS were prepared as in a and stimulated with the indicated concentrations of KCl. Data are represented as mean±s.e.m. of two independent experiments (9–15 airways per group). Full size image Af enhances Ca 2+ mobilization in ASM cells Our results suggested that Af promotes AHR by augmenting ASM contraction partially through inflammation-independent mechanisms. Agonist stimulation of GPCRs induces bronchoconstriction initially by increasing cytosolic Ca 2+ levels [18] , [19] . To determine whether Af affected GPCR-evoked Ca 2+ signalling, we incubated cultured human ASM cells (HASM) with Af extract for 24 h prior to quantification of cytosolic Ca 2+ by fluorescence microscopy. Af pre-treatment led to an increase in basal cytosolic Ca 2+ in a concentration-dependent manner ( Fig. 3a ) and significantly enhanced intracellular Ca 2+ flux in response to GPCR ligands bradykinin or histamine compared with vehicle-treated cells ( Fig. 3b–e ). In contrast, vehicle and Af -treated HASM displayed similar responses to ionomycin ( Fig. 3f ), which increase cytosolic Ca 2+ through receptor-independent mechanisms. GPCR-mediated Ca 2+ mobilization is dependent on PLCβ-mediated generation of inositol 1, 4, 5-trisphosphate (Ins P3 ), which in turn stimulates Ins P3 receptors on sarcoplasmic reticulum to release Ca 2+ into the cytosol. Accordingly, we observed increased amounts of bradykinin-evoked Ins P1 (a stable metabolite of Ins P3 ) in Af -pre-treated HASM cells compared with controls ( Fig. 3g ). 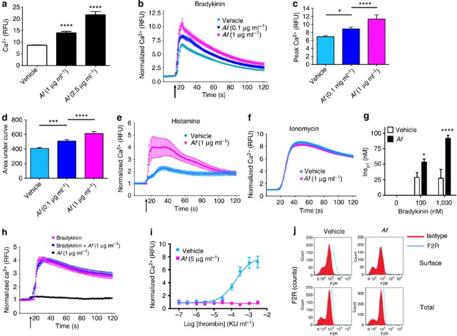Figure 3:Afmodulates Ca2+mobilization in ASM cells. Serum-starved HASM cells were left untreated or pre-incubated withAfextract for 24 h prior to measurement of cytosolic Ca2+by fluorescence microscopy as outlined in the Methods. (a) Baseline Ca2+levels after treatment are shown as mean±s.e.m. of a minimum of 60 cells per condition measured in three independent experiments (****P<0.0001, one-way analysis of variance (ANOVA)). (b–f) Agonist-induced Ca2+mobilization. Line graphs inb(bradykinin, 100 nM),e(histamine, 10 μM) andf(ionomycin, 2 μM) show normalized Ca2+measurements over time (mean±s.e.m. of 16–80 cells measured in 2–3 independent experiments) at baseline and following addition of agonist (arrows). (c) Peak and area under curve (d) of Ca2+spikes inbwere calculated (*P=0.03, ***P=0.0005 ****P<0.0001, one-way ANOVA). (g) Serum-starved HASM cells were pre-treated with vehicle orAf(2 μg ml−1) for 24 h. Accumulation of InsP1was measured after addition of the indicated concentrations of bradykinin. Data are represented as mean±s.e.m. of three independent experiments (*P=0.04, ***P<0.0001, two-way ANOVA). (h) HASM cells were stimulated acutely withAf, bradykinin (100 nM) orAf+bradykinin (100 nM) followed by measurement of Ca2+by microscopy as inb–f. Graph represents mean±s.e.m. of 7–60 cells per condition. (i) HASM cells were pre-treated with vehicle orAf(5 μg ml−1) for 24 h followed by stimulation with thrombin and measurement of Ca2+mobilization by fluorimetry. Normalized Ca2+values are represented as mean±s.e.m. of a single experiment representative of two independent experiments. (j) Surface and total F2R receptor expression in vehicle orAf-treated HASM cells was measured by flow cytometry. Representative histograms from two to three independent experiments are shown. Figure 3: Af modulates Ca 2+ mobilization in ASM cells. Serum-starved HASM cells were left untreated or pre-incubated with Af extract for 24 h prior to measurement of cytosolic Ca 2+ by fluorescence microscopy as outlined in the Methods. ( a ) Baseline Ca 2+ levels after treatment are shown as mean±s.e.m. of a minimum of 60 cells per condition measured in three independent experiments (**** P <0.0001, one-way analysis of variance (ANOVA)). ( b – f ) Agonist-induced Ca 2+ mobilization. Line graphs in b (bradykinin, 100 nM), e (histamine, 10 μM) and f (ionomycin, 2 μM) show normalized Ca 2+ measurements over time (mean±s.e.m. of 16–80 cells measured in 2–3 independent experiments) at baseline and following addition of agonist (arrows). ( c ) Peak and area under curve ( d ) of Ca 2+ spikes in b were calculated (* P =0.03, *** P =0.0005 **** P <0.0001, one-way ANOVA). ( g ) Serum-starved HASM cells were pre-treated with vehicle or Af (2 μg ml −1 ) for 24 h. Accumulation of Ins P1 was measured after addition of the indicated concentrations of bradykinin. Data are represented as mean±s.e.m. of three independent experiments (* P =0.04, *** P <0.0001, two-way ANOVA). ( h ) HASM cells were stimulated acutely with Af , bradykinin (100 nM) or Af +bradykinin (100 nM) followed by measurement of Ca 2+ by microscopy as in b – f . Graph represents mean±s.e.m. of 7–60 cells per condition. ( i ) HASM cells were pre-treated with vehicle or Af (5 μg ml −1 ) for 24 h followed by stimulation with thrombin and measurement of Ca 2+ mobilization by fluorimetry. Normalized Ca 2+ values are represented as mean±s.e.m. of a single experiment representative of two independent experiments. ( j ) Surface and total F2R receptor expression in vehicle or Af -treated HASM cells was measured by flow cytometry. Representative histograms from two to three independent experiments are shown. Full size image Addition of Af extract to HASM immediately prior to measurement of Ca 2+ concentrations (that is, without prolonged preincubation) failed to induce any Ca 2+ mobilization, and simultaneous stimulation of cells with Af extract and bradykinin did not potentiate Ca 2+ signalling induced by bradykinin alone ( Fig. 3h ). These results suggested that Af does not activate Ca 2+ signalling through a protease-activated receptor, such as F2R or F2LR1. In support of this hypothesis, we found that 24 h pre-treatment of ASM with Af actually abolished responses to thrombin and resulted in profoundly diminished levels of F2R at the plasma membrane ( Fig. 3i,j ). Thus, chronic exposure of HASM cells to Af may potentiate GPCR-evoked Ca 2+ spikes in a receptor-independent manner. Af degrades extracellular matrix Exposure of ASM cells to Af could also affect expression of receptors or elements of the excitation–contraction signalling pathway that elicit bronchoconstriction. We failed to detect increased expression of contraction-inducing receptors or intracellular contractile proteins in HASM following Af treatment ( Supplementary Fig. 1a ). However, incubation with Af induced profound changes in HASM cell morphology, including elongation and detachment, disassembly of vinculin-rich focal adhesions (adhesomes), reduced actin stress fibres ( Fig. 4a,b ) and haptotaxis ( Supplementary Movies 1 , 2 ), without altering vinculin expression ( Supplementary Fig. 1b ) or eliciting changes in cell viability, apoptosis or proliferation ( Supplementary Fig. 2 ). These results suggested that Af perturbs integrin-mediated extracellular matrix (ECM) attachments of HASM. 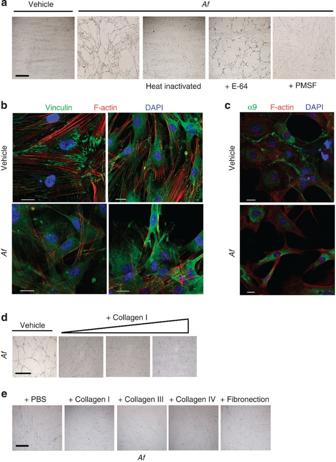Figure 4:Afserine protease activity induces morphological changes in ASM cells. (a) Serum-starved HASM cells were treated with vehicle, unmodifiedAf(5 μg ml−1), HI-AforAfincubated with PMSF (250 μM) or E-64 (10 μM) protease inhibitors. Scale bar, 200 μm; original magnification, 10 × . (b,c) Serum-starved HASM cells (b) or mouse ASM cells (c) were treated with vehicle orAf(5 μg ml−1) for 24 h. Fixed cells were stained with phalloidin (red) and anti-vinculin antibody (green) (b) or α9-integrin antibody (green) (c). Nuclei were counterstained with DAPI. Images in (b,c) are from a single experiment representative of 2-3 similar experiments. Scale bar, 20 μm; original magnification, 63 × . (d) HASM cells were cultured on plates coated with collagen I (0.2–1 mg ml−1) followed by treatment withAf(5 μg ml−1) for 48 h. DIC images are from a single experiment representative of three similar experiments. Scale bar, 200 μm; original magnification, 10 × . (e) HASM cells were seeded on plates coated with collagen I (1 mg ml−1), collagen III (0.1 mg ml−1), collagen IV (0.5 mg ml−1) or fibronectin (0.1 mg ml−1). After serum starvation, cells were treated withAf(5 μg ml−1) and visualized by microscopy 48 h post treatment. Scale bar, 200 μm; original magnification, 10 × . Images are from a single experiment representative of two to four independent experiments. Figure 4: Af serine protease activity induces morphological changes in ASM cells. ( a ) Serum-starved HASM cells were treated with vehicle, unmodified Af (5 μg ml −1 ), HI- Af or Af incubated with PMSF (250 μM) or E-64 (10 μM) protease inhibitors. Scale bar, 200 μm; original magnification, 10 × . ( b , c ) Serum-starved HASM cells ( b ) or mouse ASM cells ( c ) were treated with vehicle or Af (5 μg ml −1 ) for 24 h. Fixed cells were stained with phalloidin (red) and anti-vinculin antibody (green) ( b ) or α9-integrin antibody (green) ( c ). Nuclei were counterstained with DAPI. Images in ( b , c ) are from a single experiment representative of 2-3 similar experiments. Scale bar, 20 μm; original magnification, 63 × . ( d ) HASM cells were cultured on plates coated with collagen I (0.2–1 mg ml −1 ) followed by treatment with Af (5 μg ml −1 ) for 48 h. DIC images are from a single experiment representative of three similar experiments. Scale bar, 200 μm; original magnification, 10 × . ( e ) HASM cells were seeded on plates coated with collagen I (1 mg ml −1 ), collagen III (0.1 mg ml −1 ), collagen IV (0.5 mg ml −1 ) or fibronectin (0.1 mg ml −1 ). After serum starvation, cells were treated with Af (5 μg ml −1 ) and visualized by microscopy 48 h post treatment. Scale bar, 200 μm; original magnification, 10 × . Images are from a single experiment representative of two to four independent experiments. Full size image ECM activation of membrane-bound integrins elicits autophosphorylation of focal adhesion kinase (FAK), actin polymerization and assembly of a signalosome of cytoskeletal proteins including vinculin, paxillin and α-actinin, which are essential for actomyosin crossbridging and force generation [20] , [21] . Surprisingly, however, deficiency of α9β1 integrin in ASM by conditional genetic deletion of α9 ( Itga9 ) in mice resulted in spontaneous AHR [22] . We observed markedly reduced surface expression and increased cytosolic localization of α9 integrin in Af -treated cells compared with controls by immunofluorescence staining ( Fig. 4c ). Heat inactivation or preincubation of Af extract with a serine protease inhibitor prior to addition to HASM cells prevented Af -induced morphological change and detachment ( Fig. 4a ) as did pre-coating plates with exogenous ECM proteins including collagen I and fibronectin ( Fig. 4d,e ). Together, these results indicated that one or more serine proteases present in Af allergen extracts might digest ECM components to disrupt integrin-mediated attachments in ASM cells. A prior study demonstrated that a serine protease purified from Af culture supernatants degraded multiple ECM proteins, including elastin, collagen types I–III and fibronectin [23] . Hence, we found that the Af allergen extract used here reduced the collagen content of HASM cells in culture ( Fig. 5a ) and of PCLS ( Fig. 5b ) and digested several purified ECM components ( Fig. 5c,d ). We also determined whether exposure of HASM cells to Af induced production of matrix metalloproteinases (MMPs) or tissue inhibitor of metalloproteinases (TIMPs) that are expressed by HASM and could affect ECM composition [24] , [25] . Af treatment of HASM increased secretion of MMP1 and MMP3 compared with vehicle treatment, but not any of the others tested including MMP2, 8, 9, 10 or TIMPs 1, 2 and 4 ( Fig. 5e ). 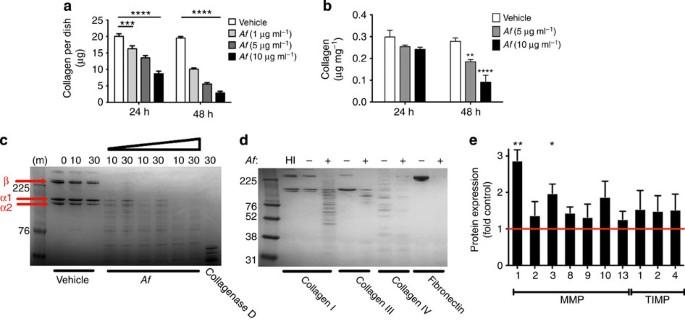Figure 5:Afdegrades the extracellular matrix. (a) Total collagen content in cultured HASM cells left untreated or incubated withAffor the indicated times. Graph shows mean±s.e.m. from a single experiment representative of three independent experiments (***P=0.006, ****P<0.0001, two-way analysis of variance (ANOVA)). (b) Collagen content in PCLS left untreated or incubated withAffor the indicated times; data are mean±s.e.m. of three independent experiments (**P=0.007; ***P<0.0001, two-way ANOVA). (c) Vehicle,Af(5, 10 or 20 μg) or collagenase D (50 μg) was incubated with collagen I (20 μg) for the indicated times at 37 °C. Samples were resolved by SDS–PAGE and visualized by Coomassie staining. α1, α2 and β subunits of collagen I are denoted by red arrows. (d) Vehicle,Af(20 μg ml−1) or heat-inactivatedAf(HI-Af, 20 μg ml−1) were incubated with collagens I, III, IV or fibronectin (20 μg) for 30 min at 37 °C. (e) Secretion of MMPs and TIMPs in cell supernatants was measured by antibody array. Bar graph depicts relative expression (mean±s.e.m. of three independent experiments) inAf-treated HASM cells compared with control (**P=0.003, *P=0.01,t-test). Figure 5: Af degrades the extracellular matrix. ( a ) Total collagen content in cultured HASM cells left untreated or incubated with Af for the indicated times. Graph shows mean±s.e.m. from a single experiment representative of three independent experiments (*** P =0.006, **** P <0.0001, two-way analysis of variance (ANOVA)). ( b ) Collagen content in PCLS left untreated or incubated with Af for the indicated times; data are mean±s.e.m. of three independent experiments (** P =0.007; *** P <0.0001, two-way ANOVA). ( c ) Vehicle, Af (5, 10 or 20 μg) or collagenase D (50 μg) was incubated with collagen I (20 μg) for the indicated times at 37 °C. Samples were resolved by SDS–PAGE and visualized by Coomassie staining. α1, α2 and β subunits of collagen I are denoted by red arrows. ( d ) Vehicle, Af (20 μg ml −1 ) or heat-inactivated Af (HI- Af , 20 μg ml −1 ) were incubated with collagens I, III, IV or fibronectin (20 μg) for 30 min at 37 °C. ( e ) Secretion of MMPs and TIMPs in cell supernatants was measured by antibody array. Bar graph depicts relative expression (mean±s.e.m. of three independent experiments) in Af -treated HASM cells compared with control (** P =0.003, * P =0.01, t -test). Full size image Notably, we detected substantially less protease activity in extracts of another common allergen, HDM, than in Af solutions with equivalent protein concentrations. HDM extract induced morphological changes and detachment of HASM cells only at much higher concentrations than did active Af , and these effects were abolished by addition of cysteine protease inhibitors ( Supplementary Fig. 3 ). Af modifies Ca 2+ signalling in ASM cells Integrin-mediated ECM interactions and the formation of focal adhesion plaques may affect the metabolism of membrane phospholipids that mediate GPCR-induced Ca 2+ spikes. Deletion of integrin α9 in mouse smooth muscle increased production of phosphatidylinositol 4,5-bisphosphate (Ins(4,5) P2 or PIP2), which is the principal substrate of PLCβ [22] . Integrin activation and FAK phosphorylation also activate Rho GTPase activating protein (p190RhoGAP), a negative regulator of RhoA activity. RhoA-associated coiled-coil forming kinase (ROCK) in turn activates phosphatidylinositol 4-phosphate 5-kinases (PIP5K), a group of enzymes that catalyze the production of PIP2. We detected increased Ins P3 in HASM cells incubated with Af ( Fig. 3g ). Addition of purified ECM components (collagen I) to HASM cultures significantly reduced Af -evoked augmentation of Ca 2+ transients ( Fig. 6a–c ), suggesting that dysregulation of cell-ECM contacts by Af protease activity increased GPCR-induced Ins P3 production. Incubation of HASM with Af abolished FAK autophosphorylation ( Fig. 6d ) and increased both basal and bradykinin-induced RhoA activation compared with vehicle-treated cells ( Fig. 6e,f ). Consequently, cellular PIP2 levels were increased in Af -treated cells compared with controls ( Fig. 6g ). Thus, increased availability of PIP2 substrate may contribute to the enhanced agonist-induced Ins P3 production and Ca 2+ mobilization we observed following Af treatment. 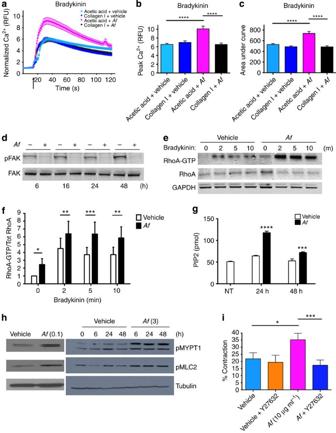Figure 6:Afenhances Ca2+sensitivity in ASM downstream of FAK and ROCK. (a–c) HASM cells were seeded on tissue culture plates pre-coated with vehicle (acetic acid) or collagen I (50 μg ml−1). Serum-starved cells were treated with vehicle orAf(1 μg ml−1) for 24 h. Cytosolic calcium was measured in individual cells following bradykinin stimulation as inFig. 3. Data are represented as mean±s.e.m. of 80–100 cells from 2 individual donors measured in 2 independent experiments (**P<0.01, ***P<0.001, one-way analysis of variance (ANOVA)). (d) HASM cells were treated with vehicle orAf(2 μg ml−1) for the indicated times followed by assessment of FAK phosphorylation and expression by immunoblotting. (e,f) HASM cells were treated with vehicle orAf(2–3 μg ml−1) followed by stimulation with bradykinin (1 μM) for the indicated times. GTP-bound and total RhoA were assessed by pull-down assay, immunoblotting and ELISA. Bar graph data are represented as mean±s.e.m. of eight experiments (*P=0.04, **P<0.008; ***P=0.0007, two-way ANOVA). (g) Serum-starved HASM cells were pre-treated with vehicle orAf(2 μg ml−1) for the times indicated. PIP2 concentrations in cell extracts were determined by ELISA. Data are represented as mean±s.e.m. of three independent experiments (***P<0.001, ****P<0.0001, one-way ANOVA). (h) HASM cells were pre-treated with vehicle orAf(0.1–3 μg ml−1) for the times indicated. MYPT1 and MLC2 phosphorylation was assessed in whole-cell lysates by immunoblotting. Blots are from a single experiment representative of three to six independent experiments. (i) Mouse PCLS were pre-treated with vehicle orAf(10 μg ml−1) for 24 h. Slices were treated with vehicle or ROCK inhibitor (Y27632, 10 μM) 1 h prior to stimulation with CCh (100 nM) and measurement of airway contraction. Data are represented as mean±s.e.m. of 2 independent experiments using 4 mice in each (16–20 airways per condition; *P=0.03, **P=0.003, one-way ANOVA). Figure 6: Af enhances Ca 2+ sensitivity in ASM downstream of FAK and ROCK. ( a – c ) HASM cells were seeded on tissue culture plates pre-coated with vehicle (acetic acid) or collagen I (50 μg ml −1 ). Serum-starved cells were treated with vehicle or Af (1 μg ml −1 ) for 24 h. Cytosolic calcium was measured in individual cells following bradykinin stimulation as in Fig. 3 . Data are represented as mean±s.e.m. of 80–100 cells from 2 individual donors measured in 2 independent experiments (** P <0.01, *** P <0.001, one-way analysis of variance (ANOVA)). ( d ) HASM cells were treated with vehicle or Af (2 μg ml −1 ) for the indicated times followed by assessment of FAK phosphorylation and expression by immunoblotting. ( e , f ) HASM cells were treated with vehicle or Af (2–3 μg ml −1 ) followed by stimulation with bradykinin (1 μM) for the indicated times. GTP-bound and total RhoA were assessed by pull-down assay, immunoblotting and ELISA. Bar graph data are represented as mean±s.e.m. of eight experiments (* P =0.04, ** P <0.008; *** P =0.0007, two-way ANOVA). ( g ) Serum-starved HASM cells were pre-treated with vehicle or Af (2 μg ml −1 ) for the times indicated. PIP2 concentrations in cell extracts were determined by ELISA. Data are represented as mean±s.e.m. of three independent experiments (*** P <0.001, **** P <0.0001, one-way ANOVA). ( h ) HASM cells were pre-treated with vehicle or Af (0.1–3 μg ml −1 ) for the times indicated. MYPT1 and MLC2 phosphorylation was assessed in whole-cell lysates by immunoblotting. Blots are from a single experiment representative of three to six independent experiments. ( i ) Mouse PCLS were pre-treated with vehicle or Af (10 μg ml −1 ) for 24 h. Slices were treated with vehicle or ROCK inhibitor (Y27632, 10 μM) 1 h prior to stimulation with CCh (100 nM) and measurement of airway contraction. Data are represented as mean±s.e.m. of 2 independent experiments using 4 mice in each (16–20 airways per condition; * P =0.03, ** P =0.003, one-way ANOVA). Full size image ROCK also promotes ASM contraction by inhibiting myosin light chain (MLC) phosphatase through phosphorylation of its MYPT1 subunit [18] . As a result, MLC phosphorylation is enhanced, which facilitates actomyosin crossbridging and ASM contraction. Af treatment of HASM cells increased both ROCK activity (MYPT1 phosphorylation) and the basal phosphorylation of MLC ( Fig. 6h ). Finally, pre-treatment of PCLS with the ROCK inhibitor Y27632 reversed the enhanced carbachol-evoked contraction of airways in PCLS treated with Af but had little effect on contraction in vehicle-treated slices ( Fig. 6i ). This result suggests that Af mediates bronchoconstriction predominantly by augmenting ROCK-mediated Ca 2+ sensitivity in ASM cells. Alp 1 mediates Af -evoked bronchoconstriction We used ion exchange chromatography and gel filtration to identify serine protease(s) responsible for the hypercontractile ASM phenotype ( Supplementary Fig. 4 ). Mass spectrometric analysis indicated that Alp 1 was the sole serine protease present in active Af extract fractions. By estimates of recovery from purification procedures and by using quantitative immunoblotting with specific polyclonal Alp 1 antisera and purified standards, we determined that Alp 1 accounted for ∼ 1% of the total protein in crude Af extracts (10–60 μg ml −1 ) ( Supplementary Fig. 5a,b ), indicating that Alp 1 concentrations in Af used for in vitro assays were roughly 0.001–0.1 μg ml −1 (see Figs 2 , 3 , 4 , 5 , 6 ). However, we estimate that the purified protein had only 10% of the protease activity of crude extracts containing equivalent concentrations of Alp 1, indicating substantial loss of protease activity during purification ( Supplementary Fig. 5c ). Treatment of HASM cells with purified Alp 1 induced cell detachment and elongation, and both outcomes were dependent on Alp 1 serine protease activity ( Fig. 7a ). Using the much more sensitive Ca 2+ assay, we found that incubation of HASM with purified Alp 1 at concentrations as low as 0.001 μg ml −1 significantly enhanced bradykinin-evoked Ca 2+ spikes ( Fig. 7b ). We determined whether Af protease activity was required for augmentation of HASM responses to contractile agonists and bronchoconstriction using heat-inactivated extracts. HI- Af did not enhance agonist-evoked Ca 2+ mobilization ( Fig. 7b ) or MYPT1 and MLC2 phosphorylation ( Fig. 7c ), nor did it significantly augment carbachol-evoked bronchoconstriction of airways in PCLS ( Fig. 7d ). By contrast, treatment of HASM cells with purified Alp 1 substantially increased MYPT1 and MLC phosphorylation compared with vehicle alone ( Fig. 7e ), and pre-treatment of PCLS with purified Alp 1 at concentrations as low as 0.1 μg ml −1 significantly increased carbachol-mediated airway contraction in PCLS compared with controls ( Fig. 7f ). Together, these results suggest that Alp 1 protease mediates the bronchoconstriction induced by Af crude allergenic extracts. 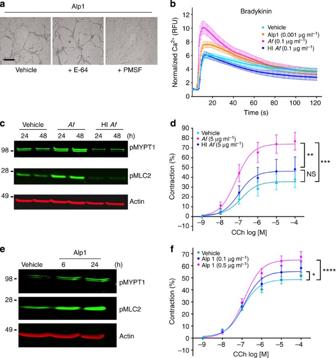Figure 7: Alp 1 serine protease regulates Ca2+sensitivity in ASM. (a) HASM cells were treated with purified Alp 1 (3 μg ml−1) in the presence or absence of serine (PMSF, 250 μM) or cysteine (E-64, 10 μM) protease inhibitors for 48 h. DIC images are from a single experiment representative of three similar experiments. Scale bar, 200 microns; original magnification, 10 × . (b) Serum-starved HASM cells were pre-incubated with vehicle, untreatedAfextract, heat-inactivatedAfor purified Alp 1 at the concentrations indicated for 24 h prior to measurement of cytosolic Ca2+in individual cells following bradykinin (100 nM) stimulation as inFig. 3. Data are represented as mean±s.e.m. of 12–25 cells from 2 individual donors measured in 2 independent experiments (P<0.0001, two-way analysis of variance (ANOVA), vehicle versusAfor Alp 1). (c) HASM cells were treated with vehicle,Afor HI-Af(3 μg ml−1) for the indicated times, and phosphorylation of MYPT1 and MLC2 was assessed by immunoblotting. Images are from a single experiment representative of three independent experiments. (d) PCLS were prepared from naïve mice and pre-treated with vehicle,Afor HI-Af(5 μg ml−1) for 24 h. Slices were stimulated with increasing concentrations of CCh and percent contraction calculated as inFig. 1. Data (mean±s.e.m.) are from a single experiment using 4 mice representative of 2 similar experiments (7–11 airways per group) fitted to a curve using the least-squares fit method.Emaxwas compared between groups by extra sum-of-squareF-test; NS, not significant (**P=0.001; ****P<0.0001, two-way ANOVA). (e) HASM cells were treated with vehicle or Alp 1 (1 μg ml−1) for the indicated times, and phosphorylation of MYPT1 and MLC2 was assessed by immunoblotting. Images are from a single experiment representative of three independent experiments. (f) PCLS were prepared from naïve mice and pre-treated with vehicle or purified Alp 1 (0.1 or 0.5 μg ml−1) for 24 h. Slices were stimulated with increasing concentrations of CCh and analyzed as ind. Data (mean±s.e.m.) are from three experiments using 2–4 mice in each (30–80 airways per condition; *P=0.03; ****P<0.0001, two-way ANOVA). Figure 7: Alp 1 serine protease regulates Ca 2+ sensitivity in ASM. ( a ) HASM cells were treated with purified Alp 1 (3 μg ml −1 ) in the presence or absence of serine (PMSF, 250 μM) or cysteine (E-64, 10 μM) protease inhibitors for 48 h. DIC images are from a single experiment representative of three similar experiments. Scale bar, 200 microns; original magnification, 10 × . ( b ) Serum-starved HASM cells were pre-incubated with vehicle, untreated Af extract, heat-inactivated Af or purified Alp 1 at the concentrations indicated for 24 h prior to measurement of cytosolic Ca 2+ in individual cells following bradykinin (100 nM) stimulation as in Fig. 3 . Data are represented as mean±s.e.m. of 12–25 cells from 2 individual donors measured in 2 independent experiments ( P <0.0001, two-way analysis of variance (ANOVA), vehicle versus Af or Alp 1). ( c ) HASM cells were treated with vehicle, Af or HI- Af (3 μg ml −1 ) for the indicated times, and phosphorylation of MYPT1 and MLC2 was assessed by immunoblotting. Images are from a single experiment representative of three independent experiments. ( d ) PCLS were prepared from naïve mice and pre-treated with vehicle, Af or HI- Af (5 μg ml −1 ) for 24 h. Slices were stimulated with increasing concentrations of CCh and percent contraction calculated as in Fig. 1 . Data (mean±s.e.m.) are from a single experiment using 4 mice representative of 2 similar experiments (7–11 airways per group) fitted to a curve using the least-squares fit method. E max was compared between groups by extra sum-of-square F -test; NS, not significant (** P =0.001; **** P <0.0001, two-way ANOVA). ( e ) HASM cells were treated with vehicle or Alp 1 (1 μg ml −1 ) for the indicated times, and phosphorylation of MYPT1 and MLC2 was assessed by immunoblotting. Images are from a single experiment representative of three independent experiments. ( f ) PCLS were prepared from naïve mice and pre-treated with vehicle or purified Alp 1 (0.1 or 0.5 μg ml −1 ) for 24 h. Slices were stimulated with increasing concentrations of CCh and analyzed as in d . Data (mean±s.e.m.) are from three experiments using 2–4 mice in each (30–80 airways per condition; * P =0.03; **** P <0.0001, two-way ANOVA). Full size image Alp 1 is present in human and murine bronchi To determine the extent to which Alp 1 reaches the airway submucosa to induce AHR in vivo , we performed immunostaining on mouse and human lung sections with anti-Alp 1 antisera. We sensitized mice intraperitoneally with Af followed by repeated intranasal challenge with Af extracts. We detected Alp 1 in bronchial smooth muscle of mice sensitized and challenged with Af , but not in naïve mice, or in animals simply inoculated intranasally with Af for 4 h or overnight prior to lung harvest in the absence of prior sensitization ( Fig. 8a and Supplementary Fig. 5d ). We also detected Alp 1 in the lung tissue ( Fig. 8b ) and BAL fluid ( Fig. 8c ) of Af -sensitized and challenged mice by immunoblotting but not in naïve mice. Based on quantitative immunoblotting, Alp 1 concentrations in BAL fluid were ∼ 0.005 μg ml −1 ( Supplementary Fig. 5b ), suggesting that we used physiologically relevant concentrations for in vitro assays. Collectively, these results demonstrated that both the allergic inflammatory response to Af and allergen protease activity seemed to be required for Alp 1 dissemination in the bronchial submucosa in mice. 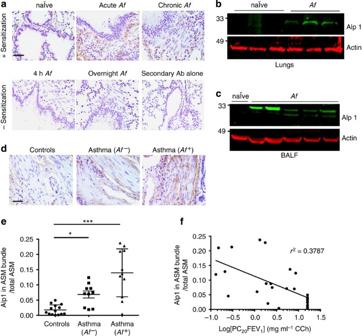Figure 8: Alp 1 is detectable in the bronchial submucosa. (a) Top panel: BALB/c mice were sensitized intraperitoneally withAfcrude extract (20 μg) mixed with 20 mg alum on days 0 and 14. Mice were challenged intranasally with PBS (‘naïve’) orAfextract (25 μg, ‘acute’) on days 25, 26 and 27, or challenged intranasally withAfextract without prior sensitization (50 μg on days 0, 7 and 14 and then with 20 μg twice per week for 4 weeks) (‘chronic’). All mice were killed 24 h after the last challenge. Bottom panel: naïve mice were challenged intranasally withAfextract (25 μg) and killed after 4 h or overnight. Alp 1 was detected using specific antisera and DAB staining of paraffin-fixed lung sections. Sections were counterstained with haematoxylin. Images are representative of four to five mice per group (Scale bar, 50 μm; original magnification, 40 × ). (b,c) Alp 1 was detected in lysates of whole-lung tissue (b) or BAL fluid (c) by immunoblotting. (d) Lung sections from healthy controls and subjects with asthma (with (Af+) and without (Af−)Afsensitivity) were immunostained with anti-Alp 1 antisera as above. Images are representative of 10–14 subjects per group (Scale bar, 50 μm; original magnification, 40 × ). (e) Alp 1 staining in the smooth muscle bundle was quantified using Image-pro Plus software and represented as the Alp 1+ASM per total ASM area (*P=0.034, ***P=0.0001, Kruskal–Wallis). (f) Correlation between the PC20FEV1 and Alp 1 staining for each subject. Figure 8: Alp 1 is detectable in the bronchial submucosa. ( a ) Top panel: BALB/c mice were sensitized intraperitoneally with Af crude extract (20 μg) mixed with 20 mg alum on days 0 and 14. Mice were challenged intranasally with PBS (‘naïve’) or Af extract (25 μg, ‘acute’) on days 25, 26 and 27, or challenged intranasally with Af extract without prior sensitization (50 μg on days 0, 7 and 14 and then with 20 μg twice per week for 4 weeks) (‘chronic’). All mice were killed 24 h after the last challenge. Bottom panel: naïve mice were challenged intranasally with Af extract (25 μg) and killed after 4 h or overnight. Alp 1 was detected using specific antisera and DAB staining of paraffin-fixed lung sections. Sections were counterstained with haematoxylin. Images are representative of four to five mice per group (Scale bar, 50 μm; original magnification, 40 × ). ( b , c ) Alp 1 was detected in lysates of whole-lung tissue ( b ) or BAL fluid ( c ) by immunoblotting. ( d ) Lung sections from healthy controls and subjects with asthma (with ( Af + ) and without ( Af − ) Af sensitivity) were immunostained with anti-Alp 1 antisera as above. Images are representative of 10–14 subjects per group (Scale bar, 50 μm; original magnification, 40 × ). ( e ) Alp 1 staining in the smooth muscle bundle was quantified using Image-pro Plus software and represented as the Alp 1 + ASM per total ASM area (* P =0.034, *** P =0.0001, Kruskal–Wallis). ( f ) Correlation between the PC 20 FEV1 and Alp 1 staining for each subject. Full size image To extend these findings to humans, we examined lung sections from control subjects or those patients with mild to moderate asthma for the presence of Alp 1. Clinical characteristics of the patient groups are summarized in Table 1 . While we detected minimal Alp 1 staining in bronchial smooth muscle bundles of lungs from healthy subjects, Alp 1 immunostaining was present in the ASM layer of lung sections from subjects with non-atopic asthma ( Fig. 8d ), and further elevated levels of Alp 1 immunoreactivity were observed in ASM of patients with asthma and Af sensitization (epicutaneous reactivity) ( Fig. 8d,e ). To evaluate the relationship between Alp 1 smooth muscle staining and AHR, we determined the provocative methacholine concentration that induced a 20% decrease in the forced expiratory volume in 1 s (PC20 FEV1 ) for each subject. There was a significant negative correlation between the amount of Alp 1 detected in the bronchial submucosa and the PC20 FEV1 ( Fig. 8f ). Table 1 Clinical characteristics of patients studied Full size table ECM composition and deposition are radically altered in both allergic and non-allergic asthma [26] , [27] , [28] . Our results suggest a novel pathophysiological mechanism whereby inflammation associated with respiratory mucosal exposure to Af allergen leads to ECM degradation through direct contact between a protease component and the bronchial submucosa. The serine protease Alp 1 secreted by Af digested ECM components directly and stimulated MMP1 release from ASM cells. We established that Alp 1 serine protease activity present in Af allergen extracts enhanced Ca 2+ sensitivity (reduced MYPT1 activity and increased MLC phosphorylation) in cultured ASM cells by disrupting integrin-dependent ASM-ECM attachments and increasing RhoA and ROCK activity. Consequently, Af failed to augment airway contraction in PCLS pre-treated with a ROCK inhibitor, suggesting that it induced bronchoconstriction primarily through pathogenic Ca 2+ sensitization. Af also evoked substantial increases in the magnitude of GPCR agonist-induced Ca 2+ transients in cultured ASM cells. We now know that intracellular Ca 2+ concentrations fluctuate repeatedly following agonist stimulation, in the form of a series of Ca 2+ oscillations [29] . The force of sustained airway contraction appears to correlate primarily with the persistence and frequency of these Ca 2+ oscillations, rather than the magnitude of the Ca 2+ spikes. However, published work has shown that while serotonin (5-HT) induced greater airway contraction of airways in PCLS than ACh, 5-HT evoked a Ca 2+ oscillation frequency that was slower than ACh in HASM cells [30] . These results suggest that the correlation between contraction and oscillation frequency depends on the agonist studied. Thus, future measurements of Ca 2+ oscillations and elucidation of the impact of Ca 2+ sensitivity (inhibition of MLCP) on the frequency-contraction relationship in PCLS will allow us to better determine the significance of our in vitro findings for bronchial contraction in vivo . How ECM–integrin interactions regulate ASM contraction in vivo also requires further study. Serine protease (elastase)-mediated airway destruction contributes to cigarette smoke-induced airway obstruction [31] . Treatment of lung slices from naïve mice with a serine protease (human neutrophil elastase) led to significantly increased airway contraction [32] . In a separate study, intratracheal administration of elastase to guinea pigs augmented bronchoconstriction in response to inhaled ACh through an unknown mechanism [33] . Although it has been argued that integrin activation by the ECM and resultant actin filament interactions at the plasma membrane promote force generation in smooth muscle cells by increasing membrane tension and cytoskeletal rigidity [20] , [21] , recent work has demonstrated that integrin signalling may regulate bronchial constriction in complex ways. For example, based on their finding that loss of α9β1 integrin in mice increased ASM contraction by stimulating PIP2 generation, Chen et al . [22] also demonstrated that addition of cell-permeable PIP2 (equivalent to the effect of Af shown here) increased carbachol-induced constriction of human airways, which was prevented by integrin-blocking antibodies. A separate study found that mice lacking the integrin-binding glycoprotein milk fat globule-EGF factor 8 (Mfge8 or lactadherin in humans), which is secreted by ASM, had exaggerated AHR following allergen challenge despite mounting an inflammatory response that was similar to control mice [34] . Their work suggested that in a physiological setting Mfge8–integrin binding in ASM served to suppress Ca 2+ sensitivity through decreased expression and activation of RhoA and ROCK. In another work, integrin–collagen I attachments were shown to promote switching of bovine tracheal smooth muscle cells towards a hyperproliferative and hypocontractile phenotype in a FAK-dependent manner [35] . Collectively, these observations are consistent with our results demonstrating that perturbation of ECM–integrin–FAK interactions by Af leads to increased RhoA and MLC activation and bronchoconstriction. Although Af protease activity was required for elicitation of maximal AHR following sensitization and challenge, our results do not exclude the possibility that allergen protease activity contributes to AHR through multiple mechanisms. Previous studies demonstrated that sensitization and intranasal challenge with purified Alp 1 alone is sufficient to induce T H 2-mediated lung inflammation and AHR [36] . Simultaneous challenge with Alp 1 purified from Af culture supernatants and a separate recombinant Af allergen ( Asp f2 ) induced a synergistic inflammatory response but did not further enhance AHR compared with challenge with Alp 1 alone. These results are consistent with our finding that Alp 1 has the capacity to affect AHR through inflammation-dependent and independent mechanisms. None of these studies addressed whether or not Alp 1 protease activity was required for the asthmatic phenotype and should be interpreted cautiously since both purified and recombinant Alp 1 have weak protease activity (the study by Moser et al . [13] and this study). Loss of activity may occur as a result of alterations in buffer pH and/or composition during purification, protein instability or the presence of endogenous activators or co-factors in the crude allergen extract. Finally, Asp f13 /Alp 1 may promote inflammation through direct effects on epithelium. Alp 1 has been shown to cause epithelial barrier dysfunction, increase Muc5ac gene expression and induce cytokine production (IL-6 and IL-8) [15] , [37] , [38] , [39] . Since respiratory exposure to Af is quite common [5] , our results indicate that an additional lung insult—allergic inflammation, a respiratory irritant or environmental exposure in the case of non-atopic disease—may be required to promote Alp 1 penetration into the bronchial smooth muscle submucosa. Several factors may account for the presence of Alp 1 (and probably other protease allergens) in the bronchial submucosa in people with asthma but not in healthy people. Recent clinical studies have demonstrated higher rates of surface airway mycosis in subjects with asthma (74%) than in controls (16%), and fungal-induced T H 2 immunity is restricted to asthma [40] . Lungs of asthmatic subjects with Af sensitivity (positive skin prick test) may be more susceptible to germination of Af spores and have a higher burden of Af recoverable from sputum [41] . Airway epithelium in subjects with asthma may be more susceptible to the permeability-inducing effects of protease allergens than that of healthy controls [11] . Taken together, these results and our work suggest that chronic pulmonary inflammation and epithelial desquamation associated with asthma promote dissemination of allergens such as Alp 1 into the bronchial smooth muscle layer. We found that extracts of another perennial allergen, HDM, contained 75% less protease activity than did Af extract at equivalent protein concentrations and did not induce ASM detachment or morphological changes similar to those elicited by Af /Alp1. As prior studies have demonstrated that HDM induces proliferation and cytokine production in ASM cells, partially through activation of F2LR1 (ref. 42 ), it is unclear whether other environmental allergens will infiltrate the bronchial submucosa and engender AHR through mechanisms equivalent to those described here. The inverse correlation between Alp 1 staining and a parameter of AHR (PC20 FEV1 ) suggests that analysis of Alp 1 in the bronchial submucosa is clinically relevant. Future studies of patients with severe asthma and/or certain disease endotypes (for example, eosinophilic versus neutrophilic inflammation) [43] may be necessary to determine whether Alp 1/ Asp f13 burden in ASM, or possibly in sputum, can be used as a biomarker to classify patients with fungal-associated asthma. Although our anti-Alp 1 antibody did not inhibit Alp 1 protease activity or protease-induced morphological changes of HASM cells ( Supplementary Fig. 6 ), Alp 1 remains a potential therapeutic target in this subset of patients pending development of an appropriate biologic. Our findings further suggest a rationale for serine protease, ROCK or PIP5K inhibitors for the treatment of specific asthma phenotypes. Reagents and antibodies Carbachol, ACh, bradykinin, histamine, ionomycin, thapsigargin, bovine serum albumin (BSA), E-64, PDGF-BB, PMSF, collagen IV, fibronectin, staurosporine and Triton X-100 were purchased from Sigma. Collagen I and III were purchased from BD Biosciences. ROCK inhibitor Y27632 was from EMD Millipore, and Collagenase D was from Roche. Methanolic Texas Red-conjugated phalloidin was obtained from Molecular Probes. Antibodies used in this study were purchased from the following sources: mouse anti-β-actin and mouse anti-vinculin (Sigma), mouse anti-GAPDH, rabbit anti-calponin, rabbit anti-SM22 and rabbit anti-B2R (Abcam), mouse anti-PLCβ (BD Biosciences), rabbit anti-ROCK1, rabbit anti-FAK, rabbit anti-pFAK Y397 (Cell Signaling Technologies), mouse anti-Rac1 and mouse anti-RhoA (Millipore). Immunoblotting and immunofluorescence HASM cells were serum starved for 48 h followed by Af pre-treatment for the indicated times. Lysates were prepared from cells, lungs or BAL fluid using radioimmunoprecipitation lysis buffer supplemented with protease inhibitor and phosphatase inhibitor cocktails (Roche) and sonication. Primary antibody staining was detected using near-infrared conjugated secondary antibodies and quantified with the LiCor Odyssey Imaging System and Image Studio software (LiCor Biosciences). For immunofluorescent staining, cells were fixed in 3.7% paraformaldehyde and permeabilized with PBS containing 0.2% vol/vol Triton X-100. Cells were then blocked in 2% (wt/vol) BSA in PBS. Cells were incubated with mouse anti-vinculin antibody (1:100) or rabbit anti-α9 integrin (Santa Cruz, 1:75) overnight at 4 °C in blocking buffer. Cells were then incubated with AlexaFluor488-conjugated goat anti-mouse or goat anti-rabbit (1:200) secondary antibody (Molecular Probes). Cells were mounted on coverglass with ProLong Gold antifade reagent with DAPI. Images were obtained using the 63 × oil immersion (numerical aperture 1.4, zoom 2) objective of a Leica SP5 confocal microscope and analyzed using Imaris software (BitPlane). Uncropped versions of the immunoblots shown in this paper are provided in Supplementary Fig. 7 . Mouse strains and asthma model Eight to ten week-old female BALB/c mice (Jackson Laboratory) were sensitized intraperitoneally with Af crude extract (Hollister-Stier) (20 μg; 1.45 × 10 −4 EU μg −1 , as determined by the ToxinSensor Chromogenic LAL Endotoxin Assay Kit (GenScript)) mixed with 20 mg Alum (Imject Alum, Pierce) on days 0 and 14. Mice were challenged intranasally with PBS (‘naïve’) or Af extract (25 μg, ‘acute’) on days 25, 26 and 27. Mice were killed 24 h after the last challenge. In some experiments, mice were treated intranasally with Af extract (25 μg) for 4 h or overnight in the absence of sensitization. Another group of mice were treated intranasally with Af extract (50 μg) on days 0, 7 and 14 and then challenged with Af extract (20 μg) twice per week for 4 weeks followed by sacrifice 24 h after last challenge (‘chronic’). All studies were performed in accordance with institutional guidelines provided by the NIAID Animal Use and Care Committee under an approved study (ASP LAD3e). Measurement of lung function in live anesthetized mice R L , was recorded using the FlexiVent system (SCIREQ Scientific Respiratory Equipment, Inc.), as described previously [44] . Analysis of lung inflammation Mouse lungs were perfused with 20 ml ice-cold PBS injected into left ventricle followed by excision and fixation in 10% neutral buffered formalin. Sections (5 μm) were prepared from paraffin-embedded lungs and stained with haematoxylin/eosin and periodic acid–Schiff. Images were obtained using a Leica DMI4000 light microscope equipped with Retiga2000R camera (QImaging, Canada) and analyzed by QCapture software. For analysis of BALF, mouse lungs were perfused with 1.5 ml ice-cold Hank's balanced salt solution, and lavage fluid was collected and centrifuged at 1,500 r.p.m. at 4 °C for 10 min. Red blood cells in the pellet were lysed by Ammonium-Chloride-Potassium lysis buffer. Total cell number was determined by haemocytometry, and differentials were determined by light microscopic examination of a Diff-Quick (Siemens)-stained cytospin (700 cells in a minimum of 15 fields at 40 × magnification). Alp 1 localization For immunostaining, mice were perfused through the left ventricle with PBS followed by lung excision and fixation in 10% neutral buffered formalin. Sections (5 μm) were prepared from paraffin-embedded lungs. Alp 1/ Asp f13 was detected by anti-Alp 1 antisera raised against a C-terminal peptide generated in rabbits (Yenzyme Antibodies LLC). Sections were counterstained with haematoxylin. Images were obtained using a Leica DMI4000 light microscope equipped with Retiga2000R camera and analyzed using QCapture software. HASM experiments HASM cells were extracted from lungs of de-identified healthy donors post-mortem obtained from the National Disease Research Interchange (NDRI) (Philadelphia, PA, USA). The isolation of ASM was performed in accordance with protocols approved by the Committee on Studies Involving Human Beings at the University of Pennsylvania. Cells were grown in Ham’s F-12 media supplemented with 10% FBS and antibiotics. Cells were seeded in 96-well plates at 10,000 cells per well. Confluent monolayers were serum starved for 48 h followed by treatment with Af or vehicle (volumetric equivalent glycerol) for the indicated times. In some experiments, Af extract was pre-incubated with PMSF (0.25 mM) or E-64 (10 μM) for 1 h at room temperature or boiled for 30 min prior to cell stimulation. Plates were coated with different ECM proteins as follows: collagens (I, III and IV) were prepared in 0.1 M acetic acid. Fibronectin was prepared in PBS. ECM proteins, PBS or 0.1 M acetic acid were incubated in wells overnight at 4 °C. Wells were then incubated with 0.2% BSA in PBS for 30 min, washed with PBS and air-dried prior to cell seeding. Video microscopy Cells were seeded on chambered coverglass slides (Lab-Tek, Nunc) and serum starved for 48 h. Differential interference contrast images were recorded every 3 min using a Leica AF6000LX confocal microscope with the 20 × dry objective. Ten fields per well were visualized for each condition 6 min before and 28 h after addition of vehicle or Af (10 μg ml −1 ). Images were analyzed and movies were recorded using Imaris software. ECM proteolytic activity assay Collagen I (20 μg) was prepared in buffer (50 mM Tris-HCl, 100 mM NaCl and 1.5 mM CaCl 2 ) and incubated with Af (20 μg) for 10 or 30 min or with collagenase D for 30 min at 37 °C. Purified collagens I, III, IV or fibronectin (20 μg) were incubated with vehicle or Af extract for 30 min at 37 °C. Samples were boiled with sample buffer at 95 °C, electrophoresed on 10% Tris-glycine gels, and visualized by Coomassie Blue staining. HASM cells or mouse PCLS were incubated with Af extract for the indicated times. Acid-pepsin soluble collagen content was measured by Sircol assay (Biocolor). MMP array Serum-starved HASM cells were treated with vehicle or Af (2 μg ml −1 ) for 24 h. Relative amounts of MMPs and TIMPs in cell supernatants were determined using a Human MMP Antibody Array (Abcam), according to the manufacturer’s instructions. Blots were developed using biotinylated primary antibodies and streptavidin and quantified using Image Studio software. Intracellular calcium measurements HASM cells were seeded at low density (30–50% confluence) onto polystyrene vessel tissue culture-treated glass slides (BD Falcon) in Ham’s F-12 medium supplemented with L -glutamine and 10% FBS for 24 h at 37 °C in 5% CO 2 . Cells were starved in serum-free medium followed by treatment with vehicle or Af extract diluted in serum-free medium for 24 h at 37 °C. F-12 media was replaced with 1:3 Fluo-8 (100 μl per chamber; Abcam Fluo-8 No Wash Calcium Assay Kit) in Ham’s F-12 media. Cells were incubated in Fluo-8 solution for 30 min then at room temperature in the dark for 30 min. Optical imaging (Nikon Eclipse TE2000-U Inverted Research Microscope) was performed immediately after the final incubation. Bradykinin (100 nM), histamine (10 μM), ionomycin (2 μM) or thapsigargin (100 nM) was added manually to the imaged chamber after 10 frames had been recorded, and images were recorded every second for 120 s. Mean, maximum and minimum grayscale measurements were obtained for a cytoplasmic region of interest (ROI) for each responding cell in each frame using FIJI [18] . Mean grayscale measurements were adjusted for background and divided by the first frame. Results were plotted as mean normalized relative fluorescence units (fold basal)±s.e.m. versus time in seconds. In Fig. 3i , intracellular Ca 2+ was measured in response to thrombin in cells plated in 96-well plates by fluorimetry as previously described [6] . Ins P1 measurements HASM cells were seeded in 96-well plates and starved in serum-free media for 48 h followed by 24 h pre-treatment with vehicle or Af (2 μg ml −1 ). Cells were then stimulated with increasing concentrations of bradykinin for 2 min. Ins P1 concentrations were measured by enzyme-linked immunosorbent assay (ELISA) as described by the manufacturer (IP-One ELISA, Cisbio Bioassays). PI(4,5)P 2 ELISA assay HASM cells were seeded in 6-cm dishes and starved in serum-free media for 48 h followed by pre-treatment with vehicle or Af (2 μg ml −1 ) for indicated times. Extraction of PI(4,5)P 2 -rich fractions and competitive ELISA assay were performed according to the manufacturer’s instructions (Echelon Biosciences, kit# K-4500). RhoA-GTP activation assay HASM cells grown in 10-cm dishes were pre-treated with Af (2 μg ml −1 ) for 24 h and then stimulated with bradykinin (1 μM) for the indicated times. Cells were scraped into ice-cold MLB lysis buffer (Millipore) supplemented with NaF, Na 3 VO 4 , protease and phosphatase inhibitor cocktails. Lysates were clarified by centrifugation at 14,000 g for 5 min. Supernatants were incubated with GST-rhotekin Rho-binding domain according to the manufacturer’s instructions (Millipore). Pull downs and total cell lysates were electrophoresed on 10% Tris-glycine gels and immunoblotted with mouse anti-RhoA antibody. In a separate series of experiments, quantities of active RhoA and total RhoA were determined in cells treated as above using the appropriate G-LISA assay (Cytoskeleton). RhoA-GTP values were normalized to total RhoA for each sample. ROCK and MLC activation assay Cells were seeded onto CellStar tissue culture plates and grown to confluence in Ham’s F-12 media supplemented with L -glutamine and 10% FBS at 37 °C in 5% CO 2 . Cells were starved in serum-free media for 72 h at 37 °C in 5% CO 2 , then treated with vehicle, Af extract or purified Alp 1 diluted in serum-free medium for 24 h. Lysates were prepared in radioimmunoprecipitation buffer and immunoblotted using the following primary antibodies: anti-pMYPT1 (T696) (Millipore), anti-pMLC2 (S18T19) (Cell Signaling Technologies) and anti-tubulin (Cell Signaling Technologies). The following secondary antibodies were used: donkey anti-mouse (Jackson ImmunoResearch Laboratories), peroxidase-conjugated or near-infrared dye-conjugated anti-mouse IgG or donkey anti-rabbit (Cell Signaling Technologies). Immunoblots were visualized using standard chemiluminescence protocols or using an Odyssey near-infrared imager (LiCor Biosciences). Flow cytometry Serum-starved HASM cells were treated with Af (5 μg ml −1 ) for 24 h and then detached from the plate using a non-enzymatic solution (Cellstripper, Corning). For surface staining of F2R, cells were incubated with PE-conjugated mouse anti-F2R (1:15, R&D Systems) or the PE-conjugated isotype control (IgG2b 1:15) for 20 min in FACS buffer at 4 °C. Cells were then fixed in PBS containing 1% paraformaldehyde. For intracellular staining, cells were fixed and permeabilized in PBS containing 0.1% saponin and 0.05% BSA prior to staining. Fluorescence data were collected using an LSRII flow cytometer (BD Biosciences) and analyzed with Flowjo software (Tree Star, Inc., Ashland, OR, USA). Precision-cut lung slice airway contraction Isolation and contraction of mouse PCLS were performed exactly as previously described with minor modifications [6] . After overnight incubation in serum-free medium, slices were treated with Af or vehicle for 24 h. The next day, slices were washed with serum-free medium and used for the contraction assay. Images were obtained using a Leica DMI4000 light microscope equipped with Retiga2000R camera and analyzed using Image-pro Plus software (Media Cybernetics). Immunohistochemistry De-identified human lung specimens and clinical parameters were obtained from the Respiratory Health Network Tissue Bank of the Fonds de recherché québécois en santé, IUCPQ site ( www.tissuebank.ca ). The IUCPQ Ethics Committee approved the collection of tissue samples by the tissue bank and their use for these studies. All subjects gave informed consent for the tissue sampling and future use of samples for research purposes. Subjects with asthma were classified as having mild to moderate asthma based on criteria established by the Global Initiative for Asthma (GINA). Human and mouse lung sections were deparaffinized and incubated with anti-Alp 1 rabbit antisera (1:1,500) followed by DAB staining and haematoxylin counterstaining. In Image-pro Plus software, the Alp 1 positive pixels within ASM bundles were chosen using the ‘Segmentation’ tool, and their area was measured by ‘Count and Measure Objects’ tool and then normalized to the total ASM bundle area. Protease activity assay Protease activity was assessed using the Fluoro Protease Assay kit (G-Biosciences) according to the manufacturer’s instructions with minor modifications. Briefly, samples were diluted into 0.1 M Tris-HCl, pH 8.0 and added to wells of a 96-well black clear bottom Costar plate. FITC-conjugated casein assay substrate (100 μl (1 μg) diluted in 0.1 M Tris-HCl, pH 8.0) was added and incubated at room temperature for 30 min. Fluorescence intensity was determined using a Tecan Infinite M200 fluorescent reader at excitation/emission of 488/530 nm. Buffer without protease was used as a blank for background subtraction. Purification of Alp 1 from Af extracts Af crude extract (50 ml) was diluted in 25 mM acetic acid (200 ml) and applied to a HiPrep CM FF 16/10 column (GE Healthcare Bioscience) pre-equilibrated with 25 mM NaOAC-HAc, pH 4.8, with a peristaltic pump at 4 °C. The column was then attached to an AKTA chromatographic system. After initial washing with equilibration buffer, bound proteins were eluted with a NaCl gradient (0–0.5 M NaCl) and fractions were collected and kept on ice. Aliquots of each fraction (1 μl) were analysed for protease activity as above. Proteolytically active fractions were combined and diluted with equilibration buffer then applied to two coupled HiTrap CM FF columns (GE Healthcare Bioscience) at 4 °C. The coupled HiTrap CM FF columns were then attached to the AKTA chromatographic system and eluted with 0–0.5 M NaCl. Protease activity of each fraction was reanalyzed, and active fractions were combined and concentrated using Amicon Ultra-4 Centrifugal Filters (Millipore) by centrifugation in a tabletop centrifuge (2,350 × g ) for each run. The concentrated fraction ( ∼ 400 μl final volume) was applied to two column-coupled Superdex 75 10/300GL columns. The columns were pre-equilibrated with 25 mM NaOAc-HAc buffer, pH 4.8, and eluted with same buffer. The fractions were collected and re-analysed for protease activity. The final active fractions were combined and the purity was determined by SDS–PAGE. Bands detected by Coomassie blue staining of SDS–PAGE gels were excised and subjected to mass spectrometric protein identification. Mass spectrometry and protein identification Identification of all SDS–PAGE separated proteins was performed on reduced and alkylated, trypsin-digested samples prepared by standard mass spectrometry protocols. The supernatant and two washes (5% formic acid in 50% acetonitrile) of the gel digests were pooled and concentrated by speed vacuum centrifugation (Labconco) to dryness directly in 200 μl polypropylene auto-sampler vials (Sun Sri, Rockwood, TN). Recovered peptides were re-suspended in 5 μl of Solvent A (0.1% formic acid, 2% acetonitrile and 97.9% water). Prior to mass spectrometry analysis, the re-suspended peptides were chromatographed directly on column, without trap cleanup. The bound peptides were separated using AQ C18 reverse phase media (3 μm particle size and 200 μm pore; 500 nl per min generating 80–120 bar pressure) packed in a pulled tip, nano-chromatography column (0.1 mm ID × 150 mm l) from Precision Capillary Columns. Chromatography was performed in-line with an LTQ-Velos Orbitrap mass spectrometer (ThermoFisher Scientific), and the mobile phase consisted of a linear gradient prepared from solvent A and solvent B (0.1% formic acid, 2% water and 97.9% acetonitrile) at room temperature. Nano LC–MS (liquid chromatography–tandem mass spectroscopy (LC–MS/MS)) was performed with a ProXeon Easy-nLC II multi-dimensional liquid chromatograph and temperature controlled Ion Max Nanospray source (ThermoFisher Scientific) in-line with the LTQ-Velos Orbitrap mass spectrometer. Computer-controlled data-dependent automated switching to MS/MS by Xcalibur 2.1 software was used for data acquisition and provided peptide sequence information. Data processing and databank searching were performed with PD 1.2 and Mascot software (Matrix Science). Data were searched against protein sequences deposited in the National Center for Biotechnology Information non-redundant protein database (NCBInr, 04/2011) and a reverse sequence decoy database. Proteins were identified using a 1% false discovery rate cutoff and two peptides per protein minimum. Cell viability assay HASM cells were seeded in 96-well plates and serum starved for 48 h. Cells were treated with vehicle, Af (5 μg ml −1 ) or HI Af . The metabolic activity of cells was measured using CellTiter-Glo Luminescent Cell Viability Assay (Promega). AnnexinV/propidium iodide staining HASM cells were seeded in four-well chamber slides (Lab-Tek, Nunc) and serum starved for 48 h. Cells were left untreated or treated with vehicle, Af (5 μg ml −1 ) for 48 h or with staurosporine (1 μM) for 6 h. Cells were then stained with FITC-conjugated Annexin V-antibody and propidium iodide as described by the manufacturer (BD Biosciences). Images were obtained using a Leica DMI4000 Fluorescence microscope equipped with Retiga2000R camera and analyzed using Image-pro Plus software. Caspase 3/7 activity HASM cells were seeded in 96-well plates, serum starved for 48 h and treated with vehicle, Af (5 μg ml −1 ) or HI Af or staurosporine (1 μM). Caspase 3/7 activity was measured by luminescence assay as an indicator of apoptosis as described by the manufacturer (Caspase-Glo 3/7 Assay, Promega). EdU staining HASM cells were seeded in four-well chamber slides (Lab-Tek, Nunc). Cells were serum starved for 48 h and left untreated or treated with vehicle, Af (5 μg ml −1 ) or PDGF (50 ng ml −1 ) for 48 h. 5-ethynyl-2′-deoxyuridine (EdU) incorporation was measured using the Click-iT EdU Imaging Kit (Molecular Probes) by microscopy on coverglass slides mounted with ProLong Gold antifade reagent with DAPI. Statistical analysis GraphPad Prism software was used for data analysis. Statistical significance was determined using student’s t -test (for two groups) or one- or two-way analysis of variance for multiple groups. Non-parametric Kruskal–Wallis tests were used to compare the human lung samples. P values <0.05 were considered significant. How to cite this article: Balenga, N. A. et al . A fungal protease allergen provokes airway hyper-responsiveness in asthma. Nat. Commun . 6:6763 doi: 10.1038/ncomms7763 (2015).